The Barbier–Grignard-type arylation of aldehydes using unactivated aryl iodides in water Carbon–carbon bond formation is the essence of organic synthesis. One of the most important methods for forming carbon–carbon bonds is the Barbier–Grignard-type reaction, which was discovered over a century ago. However, it is still highly desirable to further improve this process. In this article, we describe a Barbier–Grignard-type direct arylation of aldehydes by using unactivated iodides mediated by zinc and catalysed by rhodium in water. This method bypasses a number of challenges encountered by the conventional Barbier–Grignard reaction, such as strict exclusion of moisture and air, protection–deprotection of various acidic hydrogens in the substrates, and so forth. It thereby creates a safer, more convenient and more environmentally benign strategy to access the diarylmethanols and aryl alkyl alcohols, ubiquitous skeletons found in fine chemicals, biologically active molecules and pharmaceuticals. Importantly, the same reaction performed in an organic solvent proceeded sluggishly to give much inferior yields. It is widely recognized that the Barbier–Grignard-type reaction is one of the most important methods for forming carbon–carbon bonds and has widespread synthetic applications in modern organic chemistry [1] , [2] , [3] , [4] . Conventionally, successful handling of these reactions necessitates the strict control of anhydrous conditions, which imposes limitations on synthetic design [5] . Recently, there has been increasing interest in the development of Barbier–Grignard-type reactions in water [6] , [7] , [8] , [9] , [10] . Many types of reactions that are traditionally conducted in organic solvents can be carried out in water with additional interesting features [9] , [10] , [11] , [12] , [13] , [14] , [15] , [16] , largely due to the inherent advantages of using aqueous organometallic reactions over those occurring in organic solvents [11] , [12] , [13] , [17] , [18] , [19] . For instance, there is the practical convenience of not having to handle inflammable and anhydrous organic solvents. The tedious protection–deprotection processes for certain acidic hydrogen-containing functional groups can be eliminated, which contributes to the overall synthetic efficiency [20] , [21] , [22] , [23] , [24] . Water-soluble compounds such as carbohydrates can be used directly without the need for derivatization, and water-soluble catalyst solutions can be used for an extended period of time, which reduces operational costs [25] . The experimental procedures may be simplified since isolation of organic products and recycling of water-soluble catalysts and other reagents can be made by simple phase separation. However, while the allylation [26] , [27] , [28] , propargylation [29] , [30] , [31] , benzylation [32] , alkynylation [33] and alkylation [34] of carbonyl compounds, along with the aldol-type reaction [35] , have been successful with various metals in water, a direct Barbier–Grignard-type carbonyl arylation with unactivated aryl halide in water has yet to be developed. This is largely due to the fact that a highly active metal is required to break a non-activated C( sp 2 )-halogen bond (as well as to react with the carbonyl once the organometallic intermediate is formed). Even if the expected intermediate is successfully generated, various competing side reactions may occur when utilizing a highly reactive metal, for example, the reduction of water, the reduction of starting materials, the hydrolysis of the organometallic intermediate and the pinacol-type coupling. Essentially, these substantial difficulties have prevented the further development of aqueous organometallic reactions onto simple aryl halides. Furthermore, based on our unsuccessful attempts in the past, we ascertained that to overcome this seemingly insurmountable dilemma, a particular balance between metal reactivity and side-product conversion must be achieved without severely compromising the yield of the desired arylation product. It would be a significant expansion of aqueous organometallic chemistry by carrying out such a daunting conversion in water. Our ongoing work in Rh-catalysed direct arylation with pre-synthesized organometallic reagents in water [36] , [37] led us to believe that this process could in fact be achieved. After numerous unsuccessful attempts, herein we describe this direct Barbier–Grignard-type arylation of aldehydes with simple unactivated aryl halides mediated by zinc in water catalysed by rhodium without prior stoichiometric formation of organometallic reagent. Initial reaction conditions exploration and optimization To test our hypothesis and identify systems capable of mediating this challenging process, we investigated the reactivity of iodobenzene ( 1a ) and 4-methylbenzaldehyde ( 2a ) under the catalysis of Rh complex in water mediated by a range of metals. 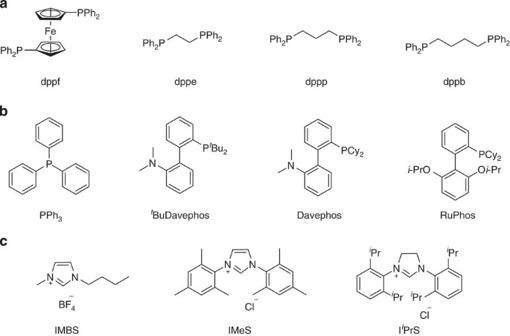Figure 1: Three categories of ligands. (a) Bidentate phosphine ligands. (b) Monodentate phosphine ligands. (c) NHC ligands. Preliminary analysis of metals, surfactants, Rh catalysts and reaction conditions ( Supplementary Table 1–3 ) revealed that a trace amount of p -methylbenzhydrol ( 3aa ) could be detected by gas chromatography–mass spectrometry from 1a and 2a with 5 mol% of [Rh(acac)(CO) 2 ], 5 mol% of dppf, 0.52 mmol of Zn in BrijC10 (2%, W/V)/H 2 O (0.5 ml) at 100 °C ( Table 1 , entry 1). Then TMEDA as additive was added and no obvious improvement was observed ( Table 1 , entry 2). Since our previous research shows that the halide is detrimental on Rh-catalysed carbonyl additions [37] , we switched the additive to 1 equivalent of NaOH and an improved reaction yield was detected ( Table 1 , entry 3). Then a range of traditional bidentate ligands ( Fig. 1a ) with different bite angles and monodentate electron-rich phosphine ligands ( Fig. 1b ) were examined, but they all failed to increase the yield of the diphenylmethanol product ( Table 1 , entries 4–10). We speculated that a more electron-donating ligand may be needed to increase the nucleophilicity of the resulting aryl-Rhodium species. The use of carbene ligand ( Fig. 1c ) led to an expected outcome distinctly displayed on gas chromatography–mass spectrometry spectra and the yield of the desired product reached 6% when I i PrS was used as the ligand ( Table 1 , entries 11–13). As the commercially available NHC ligand I i PrS exists in the form of salt, the corresponding equivalent of base is needed to deprotonate it and release the free carbene. Reducing the amount of NaOH to 7.5 mol%, surprisingly, increased the reaction yield significantly to 26% ( Table 1 , entry 14). Meanwhile, a large amount of undesired Wurtz-type byproduct from the homocoupling of iodobenzene was observed. Encouraged by this promising result, an extensive evaluation of bases, temperature, substrate ratio and halide effect [38] progressively improved conditions ( Table 1 , entries 15–20). (For expanded screening results, see Supplementary Table 4–8 ) Eventually, the optimal catalytic reactivity was achieved with [Rh(acac)(CO) 2 ] as the catalyst in combination with catalytic quantities of I i PrS and caesium pivalate in the presence of 10 mol% of LiBr in BrijC10 (2%, W/V)/H 2 O ( Table 1 , entry 20). It was worthwhile noting that the same reaction performed in an organic solvent, such as THF, MeCN and DMF, proceeded sluggishly to give the desired product but gave inferior yields. 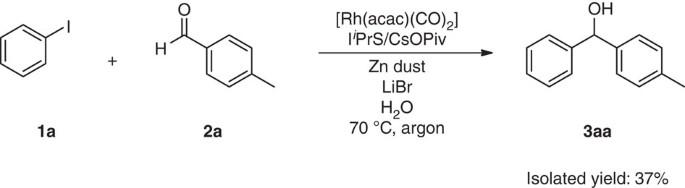Figure 4: Rhodium catalysed and zinc-mediated one-pot Barbier–Grignard-type reaction in water. The reaction proceeded smoothly in pure water and afforded a 37% isolated yield. The results revealed that the water/surfactant system was important for the activation of zinc and for scavenging the resulting alkoxide anion ( Table 1 , entries 21–23). Table 1 Selected results for optimization of the reaction conditions between iodobenzene (1a) and 4-methylbenzaldehyde (2a). * Full size table Figure 1: Three categories of ligands. ( a ) Bidentate phosphine ligands. ( b ) Monodentate phosphine ligands. ( c ) NHC ligands. Full size image Method applicability The optimized catalytic conditions ( Table 1 , entry 20) proved to be effective for the preparation of a number of substituted diphenylmethanols and aryl alkyl alcohols ( Fig. 2 ). Varying the position of methyl substituent on the benzaldehyde had little effect on the outcome of the reaction; the corresponding ortho -, meta -, and para -methylbenzhydrols were each obtained in good yields ( Fig. 2 , 3aa – 3ac ). The 4-ethyl-substituted benzaldehyde also reacted smoothly to afford the corresponding product in 70% yield ( Fig. 2 , 3ad ). In the case of benzaldehyde, the yield slightly decreased to 60% ( Fig. 2 , 3ae ). Halogen-substituted substrates, such as fluorine, chlorine and bromine, can be well tolerated in this catalytic system, giving rise to reaction yields ranging from 40–61% ( Fig. 2 , 3af – 3ah ). Notably, the tolerance of chlorine and bromine on the aromatic ring offers an opportunity for subsequent cross-coupling, facilitating expedient synthesis of highly complex biaryl molecules. For instance, the product 3ah can react with 4-acetylphenylboronic acid smoothly to afford the cross-coupling product 4ah in 75% yield when tricyclohexylphosphine was used as ligand ( Fig. 3a ). Furthermore, this Suzuki–Miyaura coupling reaction proceeded smoothly in water as well and delivered the product 4ah in 70% yield ( Fig. 3b ). Then a series of aldehydes with electron-donating and electron-withdrawing groups were found to be compatible with this protocol ( Fig. 2 , 3ai – 3an ). The reactions of the substrates with conjugate system, 4-Phenylbenzaldehyde and 1-naphthaldehyde could also proceed successfully to furnish the products in 61 and 63% isolated yields, respectively ( Fig. 2 , 3ao , 3ap ). Unexpectedly, the optimal condition can even be applied to aliphatic aldehydes (for example, n -caprylic aldehyde) and good-isolated yields can be obtained accordingly ( Fig. 2 , 3aq–3as ). Then a variety of different aryl iodides other than ortho -tolyl iodide were found to react well using this catalytic system, providing an isolated yield of up to 53% ( Fig. 2 , 3ba – 3ga ). Meanwhile, both N-(tosyl)benzylideneamine and N-benzylideneaniline were subjected to the optimized conditions. 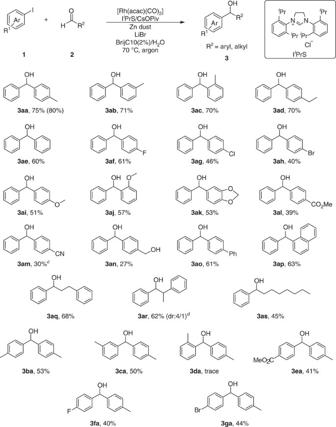However, both of them hydrolysed under the reaction condition and only diphenylmethanol 3ae was generated. Figure 2: Arylation of various aldehydesa,b. aArylation of various aldehydesaReaction conditions:1(0.6 mmol),2(0.2 mmol), Zn dust (0.78 mmol), [Rh(acac)(CO)2] (5 mol%), IiPrS (6 mol%), CsOPiv (6 mol%), LiBr 10 mol%), BrijC10 (2%, W/V)/H2O at 70 °C under argon for 24–36 h.bYield of isolated product; the1H NMR yield with 1,3,5-trimethoxybenzene as internal standard in parentheses.cThe 4-cyanobenzaldehyde dissolved in 0.5 ml of toluene was added by syringe pump at 50 °C within 18 h.dThe diastereomeric ratio (dr) (4/1) value was determined by1H NMR. Figure 2: Arylation of various aldehydes a,b . a Arylation of various aldehydes a Reaction conditions: 1 (0.6 mmol), 2 (0.2 mmol), Zn dust (0.78 mmol), [Rh(acac)(CO) 2 ] (5 mol%), I i PrS (6 mol%), CsOPiv (6 mol%), LiBr 10 mol%), BrijC10 (2%, W/V)/H 2 O at 70 °C under argon for 24–36 h. b Yield of isolated product; the 1 H NMR yield with 1,3,5-trimethoxybenzene as internal standard in parentheses. 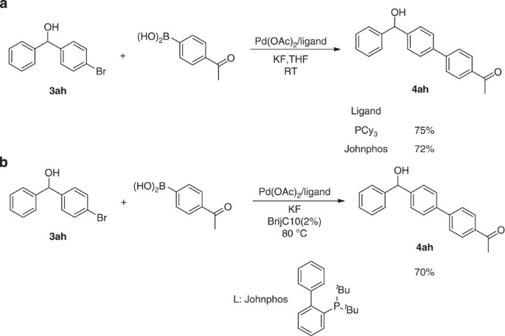c The 4-cyanobenzaldehyde dissolved in 0.5 ml of toluene was added by syringe pump at 50 °C within 18 h. d The diastereomeric ratio (dr) (4/1) value was determined by 1 H NMR. Figure 3: Suzuki–Miyaura cross-coupling. (a) The bromo-substituted product3ahcan successfully cross-couple with 4-acetylphenylboronic acid to furnish the corresponding product4ahin 75 yield. (b) Aqueous Suzuki–Miyaura cross-coupling of3ahand 4-acetylphenylboronic acid affords the product4ahin 70% yield. Full size image Figure 3: Suzuki–Miyaura cross-coupling. ( a ) The bromo-substituted product 3ah can successfully cross-couple with 4-acetylphenylboronic acid to furnish the corresponding product 4ah in 75 yield. ( b ) Aqueous Suzuki–Miyaura cross-coupling of 3ah and 4-acetylphenylboronic acid affords the product 4ah in 70% yield. Full size image Subsequently, preliminary mechanistic analysis of this transformation was performed by conducting several control experiments. It was demonstrated that the reaction could not proceed in the absence of either Rh complex or metal zinc. It clearly revealed that both Rh catalyst and metal zinc participated in this catalytic process and each performed its own function. Once the Rh catalyst and Zn work together, the reaction can proceed smoothly even without surfactant BrijC10, albeit in a low yield ( Fig. 4 ). Figure 4: Rhodium catalysed and zinc-mediated one-pot Barbier– Grignard-type reaction in water . The reaction proceeded smoothly in pure water and afforded a 37% isolated yield. Full size image In contrast to the conventional Barbier–Grignard-type reaction ( Fig. 5a ), which requires two-step strict anhydrous conditions, this method provides a more efficient and convenient one-pot approach to access the diarylmethanols and aryl alkyl alcohols ( Fig. 5c ). On the basis of our previous experience [39] and other literature studies [40] , we proposed a plausible mechanism for this transformation. We hypothesized that under certain conditions, the organometallic reagents generated in situ [41] , [42] in water could be temporarily stabilized briefly, for example organozinc reagents ( Fig. 5b ). With the assistance of transition metals such as Rh, the corresponding aryl-Rhodium species could be formed through transmetallation ( Fig. 5b , II ). Then, subsequent intermolecular addition to aldehydes could take place with scrupulous tuning of the metal catalytic centre by using various types of ligands ( Fig. 5b , III ). Finally, the expected product could be released by protonation and regenerate the active catalyst ( Fig. 5b , IV ) to close the catalytic cycle. 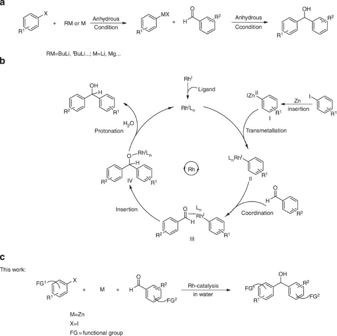Figure 5: From conventional two-step anhydrous conditions to one-pot Rh-catalysis in water. (a) Strict anhydrous conditions for the Barbier–Grignard-type reaction. Conventionally, the preformed organometal reagent (organolithium or organomagensium) reacts with carbonyl under air and moisture-free conditions to afford the corresponding product. (b) Proposed strategy for Barbier––Grignard-type carbonyl arylation in water. Entry into the catalytic cycle occurs by transmetallation of the arylmetal (organozinc) intermediate generatedin situto catalytic-active rhodium species. Coordination of carbonyl to the resulting aryl-Rhodium generates a transient intermediate, followed by insertion of the carbonyl into carbon–rhodium bond to furnish the rhodium alkoxide, which on protonation closes the catalytic cycle. (c) This work: a direct Barbier–Grignard-type arylation of aldehydes with simple unactivated aryl halides mediated by zinc and catalysed by rhodium in water. Figure 5: From conventional two-step anhydrous conditions to one-pot Rh-catalysis in water. ( a ) Strict anhydrous conditions for the Barbier–Grignard-type reaction. Conventionally, the preformed organometal reagent (organolithium or organomagensium) reacts with carbonyl under air and moisture-free conditions to afford the corresponding product. ( b ) Proposed strategy for Barbier––Grignard-type carbonyl arylation in water. Entry into the catalytic cycle occurs by transmetallation of the arylmetal (organozinc) intermediate generated in situ to catalytic-active rhodium species. Coordination of carbonyl to the resulting aryl-Rhodium generates a transient intermediate, followed by insertion of the carbonyl into carbon–rhodium bond to furnish the rhodium alkoxide, which on protonation closes the catalytic cycle. ( c ) This work: a direct Barbier–Grignard-type arylation of aldehydes with simple unactivated aryl halides mediated by zinc and catalysed by rhodium in water. Full size image In conclusion, we have succeeded in a direct Barbier–Grignard-type arylation of aldehydes with simple unactivated aryl iodides in water for the first time, the final major challenge in the field of Barbier–Grignard-type reactions in water. This method has unlocked the potential for the preparation of diarylmethanols and secondary aryl alkyl alcohols in water with good tolerance of substrate functionality. This finding should prompt more active investigation and development of aqueous organometallic reactions, which could provide a faster, safer and more environmentally friendly approach. An extension of this catalytic protocol to broaden its scope, and further mechanistic studies are in progress. Preparation of 2% BrijC10/water solution A 20 ml vial was charged with BrijC10 (200 mg), then degassed water (10 ml) was added via syringe. The mixture was then placed in a sonicator for oscillating for 10 min. Occasionally, vigorous shaking was essential for the formation of well-distributed emulsion. Then the emulsion was stored under argon. Before injecting it (2% w/v, 0.5 ml) into the reaction tube, shake it vigorously. Preparation of 4-methylbenzhydrol ( 3aa ) An oven-dried Biotage microwave tube was equipped with a magnetic stirring bar and charged with [Rh(acac)(CO) 2 ] (5 mol%), I i PrS (6 mol%), CsOPiv (6 mol%) and DCM (0.2 ml). The mixture was stirred at room temperature for 5 min and then the solvent DCM was evaporated. Zinc dust (0.78 mmol) was then loaded (and if solid, aldehyde or aryl iodide was added at this point). The tube was plugged with a rubber stopper, and then evacuated and backfilled with argon for three cycles. Under argon atmosphere, the solvent (BrijC10 in H 2 O, 2% w/v, 0.5 ml) was injected via syringe. Then iodobenzene ( 1a, 0.6 mmol, 69 μl) and 4-methylbenzaldehyde ( 2a , 0.2 mmol, 24 μl) were added. The tube was sealed and the reaction mixture was stirred at room temperature for 10 min. Then it was placed into a preheated 70 °C oil bath and the reaction mixture was stirred vigorously (1,400 r.p.m.) for 36 h. The resulting mixture was cooled to room temperature, diluted with EtOAc and filtered through a short silica gel pad. Additional EtOAc (6 × 4 ml) was needed to flush the silica gel. The above solution was concentrated under vacuum, and the residue was purified by flash chromatography on silica gel to afford 29.7 mg of the analytically pure product 3aa (ref. 36 ) (75% yield) as a liquid: thin-layer chromatography (hexane/ethyl acetate 6/1): R f =0.26; 1 H NMR (400 MHz, CDCl 3 ): δ 7.38 (d, J =7.2 Hz, 2H), 7.34 (t, J =7.2 Hz, 2H), 7.27 (d, J =8.4 Hz, 3H), 7.15 (d, J =8.0 Hz, 2H), 5.81 (s, 1H), 2.34 (s, 3H), 2.24 (br, 1H); 13 C NMR (125 MHz, CDCl 3 ): δ 143.9, 140.9, 137.3, 129.2, 128.4, 127.4, 126.5, 126.4, 76.1, 21.1. For 1 H and 13 C NMR spectra of compounds ( 3aa – 3as , 3ba – 3ga ) reported here, see Supplementary Figs 1–50 . Suzuki–Miyaura coupling of 4-bromobenzhydrol ( 3ah ) and 4-acetylphenylboronic acid An oven-dried Biotage microwave tube was equipped with a magnetic stirring bar and charged with Pd(OAc) 2 (5.0 mol%, 1.1 mg), PCy 3 (10 mol%, 2.8 mg), 4-bromobenzhydrol (0.1 mmol, 26.3 mg), 4-acetylphenylboronic acid (0.15 mmol, 25 mg) and potassium fluoride (0.33 mmol, 19.1 mg). The tube was evacuated and backfilled with argon, and THF (1.0 ml) was added through a rubber septum. The tube was then sealed and the reaction mixture was stirred at room temperature for 12 h until the 4-bromobenzhydrol had been completely consumed as judged by thin-layer chromatography analysis. The resulting mixture was filtered through a short silica gel pad and washed with ethyl acetate. The above solution was evaporated under vacuum, the residue was purified by flash chromatography on silica gel to afford the product 4ah: 22.7 mg as a white solid, yield, 75%. When the ligand Johnphos (2-biphenylyl)di- tert -butylphosphine) was utilized, a 72% of yield was obtained with all the reagents double the corresponding amounts. M.P. : 128–129 °C. 1 H NMR (400 MHz, CDCl 3 ): δ 8.02 (d, J =8.4 Hz, 2H), 7.67 (d, J =8.8 Hz, 2H), 7.61 (d, J =8.0 Hz, 2H), 7.50 (d, J =8.4 Hz, 2H), 7.43 (d, J =7.2 Hz, 2H), 7.37 (t, J =7.2 Hz, 2H), 7.32–7.29 (m, 1H), 5.92 (s, 1H), 2.63 (s, 3H); 13 C NMR (125 MHz, CDCl 3 ): δ 197.9, 145.3, 143.9, 143.6, 138.9, 135.7, 128.9, 128.6, 127.7, 127.3, 127.1, 126.5, 75.9, 26.6. MS (ESI), m / z (%): calculated for C 21 H 18 O 2 [M] 302; found [M+Na] + 325 (15%), [2M+Na] + 627 (100%); IR (neat): ν 3506, 1672, 1596, 1393, 1357, 1267, 1216, 1181, 1049, 956, 839, 799, 746, 696, 590, 517, 503; HRMS (ESI) calculated for C 21 H 18 KO 2 ([M+K] + ): 341.0938, found 341.0942. How to cite this article: Zhou, F. and Li, C.-J. The Barbier–Grignard-type arylation of aldehydes using unactivated aryl iodides in water. Nat. Commun. 5:4254 doi: 10.1038/ncomms5254 (2014).